Nanofriction in cold ion traps Sliding friction between crystal lattices and the physics of cold ion traps are so far non-overlapping fields. Two sliding lattices may either stick and show static friction or slip with dynamic friction; cold ions are known to form static chains, helices or clusters, depending on the trapping conditions. Here we show, based on simulations, that much could be learnt about friction by sliding, through, for example, an electric field, the trapped ion chains over a corrugated potential. Unlike infinite chains, in which the theoretically predicted Aubry transition to free sliding may take place, trapped chains are always pinned. Yet, a properly defined static friction still vanishes Aubry-like at a symmetric–asymmetric structural transition, found for decreasing corrugation in both straight and zig-zag trapped chains. Dynamic friction is also accessible in ringdown oscillations of the ion trap. Long theorized static and dynamic one-dimensional friction phenomena could thus become accessible in future cold ion tribology. The field of sliding friction has been recently revived because of experimental and theoretical advances especially connected with nanosystems, with brand new opportunities to grasp the underlying phenomena of this important and technologically relevant area. Unlike macroscopic friction, in which contact irregularities dominate, the nanoscale offers perfectly defined crystal lattice facets that can mutually slide. One fundamental piece of physics arising in this limit is the possibility of frictionless sliding when two perfect lattices are mutually incommensurate—their periodicities unrelated through any rational number—an idealized situation sometimes referred to as superlubric [1] . Graphite flakes sliding on graphite were, for example, shown to be pinned by static friction—the finite threshold force F s necessary to provoke motion—when aligned, but to turn essentially free sliding once a rotation makes them incommensurate [2] . An additional prediction, rigorously proven for one-dimensional (1D) infinite harmonic chains sliding in a periodic potential (the 'corrugation' potential, in frictional language), is that the incommensurate vanishing of static friction will only occur as long as the sliding chain is sufficiently hard compared with the corrugation strength. Instead, when that strength exceeds a critical value, the chain becomes locked, or 'pinned', to the corrugation, thus developing static friction despite incommensurability. Unlike most conventional phase transitions, this celebrated Aubry transition [3] , [4] , [5] , [6] involves no structural order parameter and no breaking of symmetry—just a change of phase space between the two states, the unpinned and the pinned one. The concept of pinned and unpinned states is by now qualitatively established in the sliding of real incommensurate 3D crystal surfaces [7] . Yet, the onset of static friction in the prototypical 1D chain, in which the Aubry transition is mathematically established, has never been experimentally validated. Even less is known about dynamic friction, about which we have no other insight than generic linear response [8] and some data on 3D rare gas overlayers [9] , both suggesting a quadratic increase with corrugation. Cold atomic ions can form linear chains. Despite their mutual Coulomb repulsion, ions can be corralled inside effective potential traps generated by quadrupolar radio-frequency electrodes [10] . So far, cold ion chains raised interest in view of promising applications for spectroscopy [11] , [12] , [13] , frequency standards [14] , [15] , study and control of chemical reactions [16] and quantum information [17] , [18] , [19] , [20] . We are concerned here with the possibility that they could be of use in the field of friction. In the rest of this work, explicitly simulated gedanken experiments will demonstrate that trapped cold ions may in fact represent an ideal system for future nanotribological studies addressing both static and dynamic friction. In static friction, the celebrated Aubry transition will become experimentally accessible for the first time. In dynamics, the friction rise with increasing corrugation should become measurable, giving new impulse to future theory work. Model and symmetry breaking transition The low-temperature equilibrium geometry of trapped cold ions is determined by the aspect ratio asymmetry of the confining potential, according to the effective hamiltonian [21] , [22] where r i =( x i , y i , z i ) is the position of the i th ion, m its mass, e its charge and the three terms represent kinetic energy, Coulomb repulsion and the effective parabolic trapping potential, respectively, with transverse and longitudinal trapping frequencies ω ⊥ and ω || . 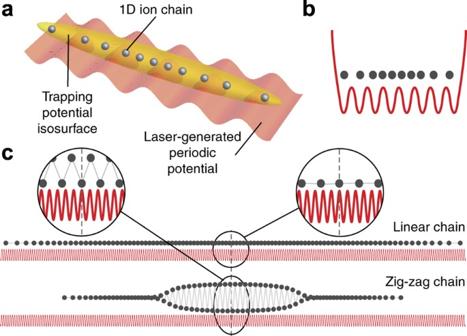Figure 1: Trapped ion chains over a periodic corrugated potential. (a,b) Sketch of the proposed ion trap configuration in a periodic potential; (c) sketch of the straight and zig-zag chain equilibrium geometries determined by different aspect ratios of the trapping quadrupolar potential. The lateral zig-zag amplitude has been artificially magnified. As is known experimentally [23] and theoretically [24] , [25] , by decreasing the asymmetry aspect ratio R = ω || / ω ⊥ , the trap potential deforms from spherical to cigar-shaped and the equilibrium ion geometry changes from 3D clusters to helices to chains, initially zig-zag and finally linear and straight along z , as shown in Figure 1c . As many as a hundred ions may be stabilized in a linear configuration, with a few μ m ion–ion spacing a 0 , typical repulsion energy e 2 / a 0 ∼ 3.3 K and temperatures below ∼ 1 μ K. An interesting observation was made by Garcia-Mata et al . [26] , that ion chains in an additional incommensurate periodic potential (produced, for example, by suitable laser beams) would, if only the spatial inhomogeneity of the trapping potential could be neglected, resemble precisely the 1D system in which an Aubry transition is expected as a function of corrugation strength. Unfortunately, the trapping potential itself introduces an additional and brutal break of translational invariance, at first sight spoiling this neat idea. The ion–ion spacing is only uniform near the chain centre, increasing strongly towards the two chain ends, where it diverges owing to the trap confinement (see, for example, Fig. 1 ). Incommensurability of the chain with the periodic potential is therefore lost, and seemingly with that all possibilities to study phenomena such as the vanishing of static friction at the Aubry transition, a transition known to depend critically on a precisely defined value of incommensurability [27] . Figure 1: Trapped ion chains over a periodic corrugated potential. ( a,b ) Sketch of the proposed ion trap configuration in a periodic potential; ( c ) sketch of the straight and zig-zag chain equilibrium geometries determined by different aspect ratios of the trapping quadrupolar potential. The lateral zig-zag amplitude has been artificially magnified. Full size image However, this conclusion is overly pessimistic. In contexts unrelated to friction, a finite chain in a periodic potential [28] , [29] , [30] is known to turn the would-be Aubry transition to a structural phase transition. The transition survives, as we will show, despite the addition of the confining trap potential. The distorted state, prevailing at strong corrugation, exhibits under suitable conditions a change of symmetry and an accompanying displacive order parameter, measuring the breaking of inversion symmetry about the chain centre. Simulations carried out by pulling the trapped chain with a longitudinal force (such as in principle provided by a static external electric field) reveal that the distortion transition is associated with a continuous onset of static friction from zero to finite, thus mimicking at finite size, and despite the trapping potential, the static friction onset theoretically expected at the ideal Aubry transition. We simulate by means of standard (weakly damped) classical molecular dynamics N =101 ions trapped by the parabolic potential of equation (1), and seek first the static ( T =0) equilibrium geometry. Below a critical aspect ratio R 0 =1.18×10 −3 , the equilibrium geometry is a linear chain, whereas at R = R 0 there is a transition to a planar partly zig-zag structure (see Fig. 1 and Supplementary Movie 1 ), further evolving to a helical structure and eventually to a 3D cluster when R →1 (ref. 24 ). Choosing R =0.5×10 −3 for the frictional simulation of a 1D trapped linear chain, we introduce an additional periodic 'corrugation' potential . To address the best-studied case of Aubry transition, we choose the corrugation wavelength λ to be 'golden ratio' incommensurate relative to the chain centre ion–ion spacing a 0 , (refs 4 , 5 ). Preserving the inversion symmetry of the chain, the periodic potential phase is chosen so that the central ion is at a potential maximum. At vanishing external force, the chain equilibrium configuration can then be followed while adiabatically increasing the corrugation amplitude U 0 . 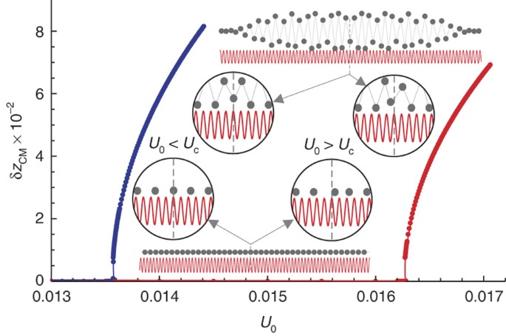Figure 2: Linear and zig-zag chain symmetry breaking. Zero-temperature ion chain equilibrium centre-of-mass coordinate δzCMversus periodic corrugation amplitudeU0for the linear chain (red) and zig-zag chain (blue). Position, time and energies in dimensionless units (seeMethods). The insets zoom on the linear chain and the zig-zag central portions, highlighting the symmetry breaking taking place atU0=Ucand above. As shown in Figure 2 , the chain ground state remains fully left–right symmetric right up to a critical corrugation amplitude U c =0.01627 (in dimensionless units; see Methods ), where it sharply turns asymmetric, with the centre of mass (CM) moving right or left by an amount δ z CM ( U 0 ) (see Supplementary Movie 2 ). This transition, similar but not identical to that known for free finite chains [28] , [30] , is the remnant of the Aubry transition of the ideal infinite chain. In both the finite and the infinite chain, the probability to find an ion (here the central ion) positioned exactly at a periodic potential maximum vanishes above the critical corrugation strength, at which the ion moves out to a minimum distance ψ away from the potential maximum [5] , [31] . Unlike the Aubry transition that has no structural order parameter, the ( T =0) finite chain transition is structural, characterized by a displacive order parameter δ z CM , Ising-like as the central ion can identically fall left or right of the centre. This order parameter grows continuously as | U 0 – U c | β at the transition (see Fig. 2 ). We find β =0.496±0.005 for the trapped linear ion chain, which is practically coincident with the exponent κ =0.5 known for finite chains with short-range forces and without trapping potential [29] . Moreover, upon reducing the confining shape asymmetry by increasing the aspect ratio to R =1.2×10 −3 , the chain equilibrium geometry evolves from linear to a partly planar zig-zag ( Fig. 2 ), still symmetric about z =0 at U 0 =0. For increasing corrugation, a symmetry-breaking transition similar to that of the linear chain takes place here too at U c =0.01357—a smaller value, as in the zig-zag the ions are further apart—and for such case β =0.504±0.005 (see Supplementary Movie 3 ). For both the linear and the zig-zag chain, the critical amplitude U c also depends on the incommensurability ratio λ / a 0 (not shown). Although these results are valid at T =0, it should be stressed that as in all small-size systems, the temperature will cancel all symmetry breaking and order parameters, owing to thermal jumps taking place above the energy barrier Δ, which separates the two opposite Ising-like order parameter valleys. However, the mean time lapse between jumps diverges exponentially when T ≪ T b ∼ Δ/ k B , the trap blocking temperature. Except too close to U c , ion traps are routinely cooled down to temperatures of order 10 −7 (in our units e 2 / d ∼ 6.3 K) way below the blocking temperature (for example, T b ∼ 180 μ K even for U 0 =0.014, barely above the critical U c =0.01357). Therefore, even at finite temperatures, the ion chain will still break inversion symmetry and exhibit a distortive order parameter for macroscopically long times similar to the T =0 results detailed above. Figure 2: Linear and zig-zag chain symmetry breaking. Zero-temperature ion chain equilibrium centre-of-mass coordinate δ z CM versus periodic corrugation amplitude U 0 for the linear chain (red) and zig-zag chain (blue). Position, time and energies in dimensionless units (see Methods ). The insets zoom on the linear chain and the zig-zag central portions, highlighting the symmetry breaking taking place at U 0 = U c and above. Full size image Determination of the static friction force Thus far the description of the ion trap in a periodic corrugation, still free of external forces. To study static friction, we apply a uniform force F , such as that of an electric field parallel to the chain axis. The usual procedure used to determine static friction—the smallest force capable of causing a pinned-to-sliding transition, following which the chain is depinned with unlimited sliding—does not work here, as the field-induced CM displacement δ z CM ( F ) is finite by necessity, owing to the confining trap potential. We circumvent that problem by monitoring another quantity, namely the restoring force F R that must be applied to the chain in order to shift its CM coordinate back exactly to zero—keeping the central ion of the chain exactly on top of the corrugation maximum at z =0. In the infinite free chain, this alternative definition of static friction coincides with the standard pinned-to-sliding Peierls–Nabarro threshold force F PN [5] , [32] , identifiable with the static friction F s of the system. In the pinned Aubry state, the critical force F PN is exactly sufficient to drive to zero the minimum equilibrium deviation ψ of one 'kink' away from the nearest corrugation maximum, eventually triggering the free motion that initiates the pinned-to-sliding transition of the whole system [5] , [33] . Analogously, for trapped ions a growing external force F gradually causes the central atom deviation from the potential maximum to decrease, and eventually to vanish at F = F R . We conclude that F R measures the static friction even in a trap, in which proper free sliding is impeded. As shown in Fig. 3 (inset), for U 0 < U c the central ion of the trap spontaneously remains precisely at zero, whence F R =0. However, at U 0 > U c , at which the force-free displacive order parameter δ z CM turns spontaneously non-zero, a finite restoring force F R must be applied in order to cancel it. The growth of the symmetry-restoring force F R with U 0 ( Fig. 3 ) is, despite the larger threshold, generally close to the Aubry static friction expected theoretically for the infinite ideal chain [1] , [4] , when calculated for same chain parameters a 0 , U 0 and golden ratio λ , as those at the trapped chain centre. We have thus established a connection between the trapped chain restoring force F R and the Peierls–Nabarro static friction of the infinite chain, of tribological significance [1] . Numerical differences between the two are of course hardly surprising. The finite size Na 0 cuts off the Aubry critical region in which the correlation length exceeds this size. For the same reason, the chain-depinning exponent χ , F R ∼ | U 0 – U c | χ , which we find to be about 1.85±0.2, differs from the higher exponent ( ∼ 3) expected for the infinite free chain for short-range forces [5] , [31] , [32] . The effective static friction of linear and zig-zag chains also differs slightly (see Fig. 3 ); the softer zig-zag chain is easier to pin, owing to its larger compliance than the linear chain. Overall, both cases provide a measurable realization of the sharp onset of static friction at the Aubry transition, valid beyond the limitations of a trapped chain. 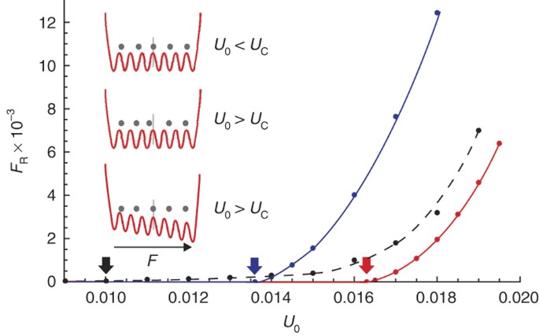Figure 3: Ion chain static friction versus corrugation amplitude. Effective static friction measured by the restoring forceFRnecessary to symmetrize the system about the centre, versus corrugation amplitudeU0for the trapped linear ion chain (red) and zig-zag chain (blue). The insets illustrate the procedure used. Black dashed line: calculated theoretical static friction at the Aubry transition of the ideal infinite golden ratio incommensurate chain. Arrows mark the vanishing point of effective static friction in each case. Figure 3: Ion chain static friction versus corrugation amplitude. Effective static friction measured by the restoring force F R necessary to symmetrize the system about the centre, versus corrugation amplitude U 0 for the trapped linear ion chain (red) and zig-zag chain (blue). The insets illustrate the procedure used. Black dashed line: calculated theoretical static friction at the Aubry transition of the ideal infinite golden ratio incommensurate chain. Arrows mark the vanishing point of effective static friction in each case. Full size image Dynamic friction Besides static friction and its Aubry-like vanishing transition, ion traps could in addition provide nontrivial insight on dynamic friction. The onset of dynamical friction in depinned infinite chains is a very subtle event, as discussed in the literature [34] ; the pinned-to-sliding onset has been simulated and elegantly described by Braun and coworkers [5] , [33] . In tribology, we are primarily interested in the growth, for incommensurate sliders at finite sliding speed, of dynamical friction with increasing corrugation. To simulate the chain dynamical behaviour, we initially displace the ions away from their equilibrium configuration with a static field, then remove the field and follow the spontaneous 'ringdown' damping of the bodily oscillation of the whole chain in the trap potential. For an initial large CM displacement of order 10 a 0 , the chain oscillation damping is readily observable, and for a weak corrugation U 0 ≪ U c can be measured even in the absence of an external heat bath. The initial potential energy (here ∼ 0.1) is converted to Joule heating of the chain at a ringdown rate, which is a direct measure of dynamic friction. Actually, a trapped chain has an intrinsic dynamic friction even in the absence of corrugation, because of the trap-potential-induced transfer of kinetic energy from the CM motion to internal chain phonon modes. 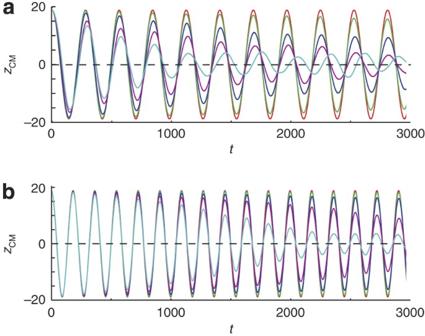Figure 4: Ion chain kinetic ringdown oscillations. The two panels show thezCMcoordinate, for the linear (a) and the zig-zag (b) chains, as a function of time for different values ofU0<Uc: redU0=0, greenU0=0.001, blueU0=0.0002, magentaU0=0.0003 and cyanU0=0.0004. However, this effect is small; the conversion and the corresponding dynamic friction is strongly enhanced by the corrugation potential, as shown in Figure 4 and in Supplementary Movies 4 and 5 (for the linear and zig-zag configurations of the chain, respectively). Simulation of the chain oscillations yields a ringdown amplitude decay for both linear and zig-zag chains, of the form A 0 exp−[ t /τ]. We find that the lifetime τ ( U 0 ) strongly decreases for increasing U 0 . The corresponding increase in dynamic friction F D , directly proportional to τ −1 , is to a good approximation quadratic, F D ∼ a+bU 0 2 for weak corrugation ( Fig. 5 ). A quadratic increase is just what the linear response theory predicts based on Fermi's golden rule [8] , [35] . It also agrees with the experimental quartz crystal microbalance monolayer friction data of Coffey and Krim [9] . 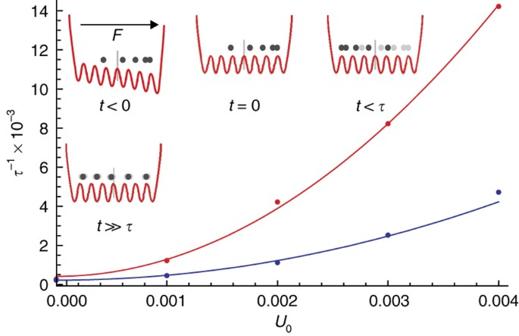Figure 5: Dynamic friction in ion chain oscillations. (a) Inverse decay timeτ−1of CM ringdown oscillations, measuring the dynamic friction of the ion chain, linear (red) and zig-zag (blue). The inset illustrates the procedure used to obtain it. Continuous lines represent fits of the forma+bU02(a=0.014 andb=867.82 for the linear chain anda=0.0 andb=250.31 for the zig-zag). There is no dynamic friction theory for the infinite linear chain to be used for comparison with the trapped chain results of Figure 5 ; therefore, the present results can be considered as a first exploratory result in this direction. The exceedingly small values of a indicate the strong harmonicity of the chain, whose CM motion can only with great difficulty excite the higher frequency intra-chain phonons in the absence of corrugation. The quadratic increase with U 0 reflects the effective opening of anharmonic excitation channels through Umklapp scattering. Larger oscillation amplitudes could not be readily simulated because the Joule heat liberated would in that case be excessive and would destroy the chain in the lack of some external dissipation mechanism. A fully nonlinear behaviour of dynamic friction would be expected to emerge in that case, with outcomes strongly dependent upon the heat disposal mechanism. Figure 4: Ion chain kinetic ringdown oscillations. The two panels show the z CM coordinate, for the linear ( a ) and the zig-zag ( b ) chains, as a function of time for different values of U 0 < U c : red U 0 =0, green U 0 =0.001, blue U 0 =0.0002, magenta U 0 =0.0003 and cyan U 0 =0.0004. Full size image Figure 5: Dynamic friction in ion chain oscillations. ( a ) Inverse decay time τ −1 of CM ringdown oscillations, measuring the dynamic friction of the ion chain, linear (red) and zig-zag (blue). The inset illustrates the procedure used to obtain it. Continuous lines represent fits of the form a + bU 0 2 ( a =0.014 and b =867.82 for the linear chain and a =0.0 and b =250.31 for the zig-zag). Full size image The remarkable static and dynamic friction properties emerging for trapped ion chains seem well amenable to experimental study. The exceedingly small values of the distortion δ z CM necessary to establish an accurate value for the effective static friction F R will require a fine tuning of corrugation and applied force. However, upon increasing the force, the instant F = F R is reached and the symmetric position δ z CM =0 is attained; the chain will spontaneously jump over the barrier to the opposite Ising order parameter valley. By, for example, alternating in time rightward and leftward forces, the effective static friction F R could become readily detectable in experiment as the threshold force magnitude for the chain's CM to sway visibly leftward and rightward. The present static friction study is conducted at zero temperature, ignoring quantum effects, without external sources of heating, cooling or damping, and assuming that a sufficiently strong effective periodic corrugation potential can be laser generated. Although each of these points requires careful consideration, none, as will be discussed below, is in our view fatal to the results presented for static friction. The proposed dynamic friction experiment would heat up the trapped ion chains and cause their destruction once the Joule heating is excessive. However, we verified that even at a temperature of ∼ 0.55 K, orders of magnitude higher than the effective chain Debye temperature of ∼ 145 μK (considering Mg + ions separated by a 0 =5 μm), the chain is still stable in the strong trapping potential. In conclusion, the field of cold atoms has had a tremendous development, recently covering important interdisciplinary areas such as Anderson localization [36] . Now it is proposed that the potential tribological impact of cold ion results could also be significant. The onset of static friction is a rich problem of current interest [37] , [38] , and so is the dynamic friction growth with corrugation [9] . Most importantly, ion chains represent a new clean design, free of most complications of real crystal lattices and with many more controllable parameters for a study of basic nanofrictional properties. Simulation details The equations of motion derived from (1) turn dimensionless by defining the quantity d 3 =e 2 / mω ⊥ 2 , and expressing distance in units of d , time in units of 1/ ω ⊥ and the mass in units of m . With this definition, energy and force are also dimensionless in units of e 2 / d and e 2 / d 2 , respectively. Simulations are carried out using classical molecular dynamics, when necessary with a weak frictional damping, and mostly at zero or low temperature. The equations of motion have been integrated using a velocity-Verlet algorithm with a time step Δ t =5×10 −3 time units. The threshold trap potential asymmetry R 0 for linear/zig-zag structure transition is determined with adiabatic increments Δ R =10 −4 starting from R =0.5×10 −3 . The critical periodic corrugation potential amplitude U c for the symmetric–asymmetric transition of linear and zig-zag chains is obtained by adiabatic increments Δ U 0 =10 −5 starting from an initial value U 0 =0.012 for the zig-zag configuration and U 0 =0.015 for the linear chain. In all the adiabatic increment procedures, a small viscous damping − γv i , with γ =0.01, is applied to all ions in order to eliminate the excess energy. With our choice of γ , a total time of 2500 units between successive increments is enough to damp all the excess energy away. Temperature and quantum effects The present study is conducted conventionally at zero temperature, ignoring quantum effects, without external sources of heating, cooling or damping, and assuming that a sufficiently strong periodic potential can be laser generated for the transition to take place at the given incommensurability provided by the laser field. Although temperature is in reality finite (typically of order 100 nK), the previously reported comparison between left and right chain distortion energies with k B T implies a symmetry-broken state lifetime much longer than any measurement time, justifying the zero temperature treatment, at which data and their significance are clearer. Moreover, in this regime, quantum zero-point effects could in principle alter some of the details close to the depinning threshold, but are otherwise not expected to affect the overall friction picture, both static and dynamic. Corrugation potential magnitude To produce the effective periodic corrugation potential, the wavelength ξ of a laser light must fit an electronic excitation in the spectrum of the chosen ion species (for example, 280 nm for Mg + , 397 nm for Ca + or 399 nm for Yb + ); with a typical a 0 =5 μ m the golden mean incommensurate periodic potential wavelength is λ =3000 nm ≫ ξ; nevertheless, the desired λ value for the effective periodic potential can be obtained by laser beam crossing at a chosen angle [26] . Experimentally, it is mandatory to realize a sufficient corrugation amplitude U = U 0 for the Aubry transition to occur. Assuming, for example, Mg + ions and golden ratio incommensurability, the critical amplitude of the effective periodic potential U c requires a laser intensity of some hundred KW/m 2 , which seems still within reach. On the other hand, the Aubry pinning transition becomes, as is well known, easier with any chain-corrugation incommensurability different from the golden ratio [27] , whereby in general the transition would occur even with weaker corrugation amplitudes than U 0 . Phase misalignment effects We assumed so far the possibility to position the corrugation potential maximum precisely at the minimum of the harmonic trap, a feat that may be experimentally difficult. Slight shifts of the corrugation potential phase away from that point would, however, simply smear the Aubry pinning onset in the same way as a weak symmetry breaking field transition would affect a phase transition. Chain heating during ringdown In the oscillation ringdown simulations, the initial potential energy difference 8.9, due to the chain displacement of 10 a 0 , is gradually converted to heating of the chain. With the mass of Mg + , the final temperature reached is ∼ 0.55 K, orders of magnitude higher than the effective chain Debye temperature of ∼ 145 μK. Despite this, we verified by direct simulation that at this temperature the chain is still stable in the strong trapping potential. How to cite this article: Benassi, A. Nanofriction in cold ion traps. Nat. Commun. 2:236 doi: 10.1038/ncomms1230 (2011).